Novel genetic loci associated with hippocampal volume The hippocampal formation is a brain structure integrally involved in episodic memory, spatial navigation, cognition and stress responsiveness. Structural abnormalities in hippocampal volume and shape are found in several common neuropsychiatric disorders. To identify the genetic underpinnings of hippocampal structure here we perform a genome-wide association study (GWAS) of 33,536 individuals and discover six independent loci significantly associated with hippocampal volume, four of them novel. Of the novel loci, three lie within genes ( ASTN2 , DPP4 and MAST4 ) and one is found 200 kb upstream of SHH . A hippocampal subfield analysis shows that a locus within the MSRB3 gene shows evidence of a localized effect along the dentate gyrus, subiculum, CA1 and fissure. Further, we show that genetic variants associated with decreased hippocampal volume are also associated with increased risk for Alzheimer’s disease ( r g =−0.155). Our findings suggest novel biological pathways through which human genetic variation influences hippocampal volume and risk for neuropsychiatric illness. Brain structural abnormalities in the hippocampal formation are found in many complex neurological and psychiatric disorders including temporal lobe epilepsy [1] , vascular dementia [2] , Alzheimer’s disease [3] , major depression [4] , bipolar disorder [5] , schizophrenia [6] and post-traumatic stress disorder [7] , among others. The diverse functions of the hippocampus, including episodic memory [8] , spatial navigation [9] , cognition [10] and stress responsiveness [11] are commonly impaired in a broad range of diseases and disorders of the brain that are associated with insults to the hippocampal structure. Further, the cytoarchitectural subdivisions (or ‘subfields’) of the hippocampus are associated with distinct functions. For example, the dentate gyrus (DG) and sectors 3 and 4 of the cornu ammonis (CA) are involved in declarative memory acquisition [12] , the subiculum and CA1 play a role in disambiguation during working memory processes [13] , and the CA2 is implicated in animal models of episodic time encoding [14] and social memory [15] . The anterior hippocampus, which includes the fimbria, CA subregions and hippocampal -amygdaloid transition area (HATA), may be involved in the mediation of cognitive processes including imagination, recall and visual perception [16] and anxiety-related behaviours [17] . Environmental factors, such as stress, affect the hippocampus [18] , but genetic differences across individuals account for most of the population variation in its size; the heritability of hippocampal volume is high at around 70% (refs 19 , 20 , 21 ). High heritability and a crucial role in healthy and diseased brain function make the hippocampus an ideal target for genetic analysis. We formed a large global partnership to empower the quest for mechanistic insights into neuropsychiatric disorders associated with hippocampal abnormalities and to chart, in depth, the genetic underpinnings of the hippocampal structure. Here we perform a GWAS meta-analysis of mean bilateral hippocampal volume in 33,536 individuals scanned at 65 sites around the world as a joint effort between the Enhancing Neuroimaging Genetics through Meta-analysis (ENIGMA) and the Cohorts for Heart and Aging Research in Genomic Epidemiology (CHARGE) consortia. Our primary goal is to find common genetic determinants of hippocampal volume with previously unobtainable power. We make considerable efforts to coordinate data analysis across all sites from both consortia to maximize the comparability of both genetic and imaging data. Standardized protocols for image analysis and genetic imputation are freely available online (see URLs). In the most powerful imaging study of the hippocampus to date, we shed light on the common genetic determinants of hippocampal structure and allow for a deepened understanding of the biological workings of the brain’s memory centre. We confirm previously identified loci influencing hippocampal volume, identify four novel loci and determine genome-wide overlap with Alzheimer's disease. Novel genome-wide markers associated with hippocampal volume Our combined meta-analysis ( n =26,814 individuals of European ancestry) revealed six independent, genome-wide significant loci associated with hippocampal volume ( Fig. 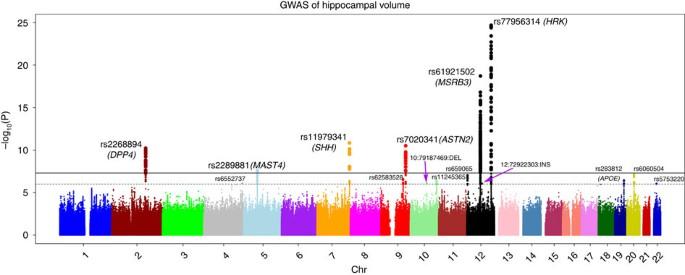Figure 1:Common genetic variants associated with hippocampal volume (N=26,814 of European ancestry). A Manhattan plot displays the associationPvalue for each single-nucleotide polymorphism (SNP) in the genome (displayed as –log10of theP-value). Genome-wide significance is shown for theP=5 × 10−8threshold (solid line) and also for the suggestive significance threshold ofP=1 × 10−6(dotted line). The most significant SNP within an associated locus is labeled. For the significant loci and age-dependent loci (Chromosome 19) we labeled the nearest gene, which is not necessarily the gene of action. 1 ; Table 1 ). Four are novel: with index SNPs rs11979341 (7q36.3; P =1.42 × 10 −11 ), rs7020341 (9q33.1; P =3.04 × 10 −11 ), rs2268894 (2q24.2; P =5.89 × 10 −11 ), and rs2289881 (5q12.3; P =2.73 × 10 −8 ). The other two loci have been previously characterized in detail: with index SNPs rs77956314 (12q24.22, P =2.06 × 10 −25 ), in linkage disequilibrium (LD) ( r 2 =0.901 in European samples from the 1000 Genomes Project, Phase 1v3) with our previously identified variant at this locus (rs7294919) and rs61921502 (12q14.3, P =1.94 × 10 −19 ), in LD ( r 2 =0.459) with previous top locus rs17178006 (refs 22 , 23 , 24 ; Fig. 2a–f ). In addition to these SNPs, we identified nine independent loci with a statistically suggestive influence on hippocampal volume ( P <1 × 10 −6 ; Supplementary Data 4 ). All pathway results and gene-based P values are summarized in Supplementary Data 6 and 7 . Figure 1: Common genetic variants associated with hippocampal volume ( N =26,814 of European ancestry). A Manhattan plot displays the association P value for each single-nucleotide polymorphism (SNP) in the genome (displayed as –log 10 of the P -value). Genome-wide significance is shown for the P =5 × 10 −8 threshold (solid line) and also for the suggestive significance threshold of P =1 × 10 −6 (dotted line). The most significant SNP within an associated locus is labeled. For the significant loci and age-dependent loci (Chromosome 19) we labeled the nearest gene, which is not necessarily the gene of action. Full size image Table 1 Genetic variants at six loci were significantly associated with hippocampal volume. 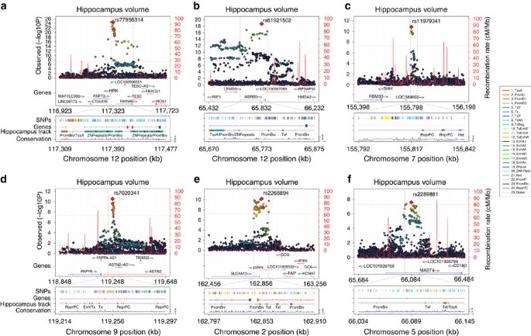Figure 2: Functional annotation within genome-wide significant loci. For each panel (a–f), zoomed-in Manhattan plots (±400 kb from top SNP) are shown with gene models below (GENCODE version 19). Plots below are zoomed to highlight the genomic region that likely harbors the causal variant(s) (r2>0.8 from the top SNP). Genomic annotations from the Roadmap Epigenomics Consortium53are displayed to indicate potential functionality (see Methods for detailed track information). Each plot was made using the LocusTrack software55(see URLs). Full size table Figure 2: Functional annotation within genome-wide significant loci. For each panel ( a – f ), zoomed-in Manhattan plots (±400 kb from top SNP) are shown with gene models below (GENCODE version 19). Plots below are zoomed to highlight the genomic region that likely harbors the causal variant(s) ( r 2 >0.8 from the top SNP). Genomic annotations from the Roadmap Epigenomics Consortium [53] are displayed to indicate potential functionality (see Methods for detailed track information). Each plot was made using the LocusTrack software [55] (see URLs). Full size image Variance explained in hippocampal volume by common variants Common variants genotyped from across the whole-genome explained as much as 18.76% (s.e. 1.56%) of the observed variance in human hippocampal volume, based on LDSCORE regression [25] ( Supplementary Fig. 3 ). Common genetic variants account for around a quarter of the overall heritability, estimated in twin studies to be around 70% (refs 19 , 20 , 21 ). Further partitioning the genome into functional categories using LDSCORE [26] revealed significant over-representation of regions evolutionarily conserved in mammals ( P =0.0026): 2.6% of the variants accounted for 43.3% of the 18.76% variance explained ( Fig. 3 ). 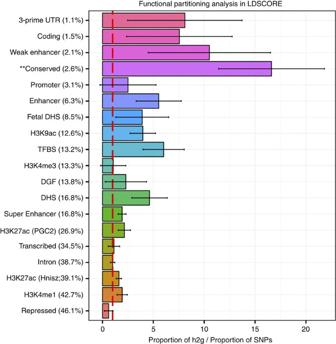Figure 3: Analysis of variance explained, functional annotation, and pathway analysis. LDSCORE regression analysis for different functional annotation26categories (described further in Finucaneet al.26). Plotted values are the proportion ofh2gexplained divided by the proportion of SNPs in a given functional category. Values are significantly over- or under-represented if they differ significantly from 1. Values are plotted with a standard error calculated with a jackknife in LDSCORE. Evolutionarily conserved regions across mammals significantly contributed to the heritability of hippocampal volume (indicated by **). Figure 3: Analysis of variance explained, functional annotation, and pathway analysis. LDSCORE regression analysis for different functional annotation [26] categories (described further in Finucane et al . [26] ). Plotted values are the proportion of h 2 g explained divided by the proportion of SNPs in a given functional category. Values are significantly over- or under-represented if they differ significantly from 1. Values are plotted with a standard error calculated with a jackknife in LDSCORE. Evolutionarily conserved regions across mammals significantly contributed to the heritability of hippocampal volume (indicated by **). Full size image Effects of top variants on hippocampal subfield volume To test for differential effects on individual subfields of the hippocampal formation, we examined the six significant variants influencing whole hippocampal volume in a large cohort ( n =5,368). We found that the top SNP from our primary analysis, rs77956314, has a broad, nonspecific effect on hippocampal subfield volumes with the greatest effect in the right hippocampal tail ( P =1.27 × 10 −8 ). rs61921502 showed strong lateral effects across right hippocampal subfields with the largest effect in the right hippocampal fissure ( P =6.45 × 10 −9 ). rs7020341 showed greatest effects bilaterally in the subiculum (left: P =1.59 × 10 −8 ; right: P =1.42 × 10 −8 ). rs2268894 show left-lateralized effects across hippocampal subfields with the strongest effect in the left hippocampal tail ( P =1.76 × 10 −5 ). The remaining two variants (rs11979341 and rs2289881) did not show significant evidence of association across any of the hippocampal subfields. The full set of results from the hippocampal subfield analysis is tabulated in Supplementary Data 8 . Genetic overlap with hippocampal volume We used LDSCORE [27] regression to quantify the degree of common genetic overlap between variants influencing the hippocampus and those influencing Alzheimer’s disease. We found significant evidence of a moderate, negative relationship whereby variants associated with a decrease in hippocampal volume are associated with an increased risk for Alzheimer’s disease ( r g =−0.155 (s.e. 0.0529), P =0.0034; see Methods). We identified six genome-wide significant, independent loci associated with hippocampal volume in 26,814 subjects of European ancestry. Of the six loci, four were novel: rs11979341 (7q36.3; P =1.42 × 10 −11 ), rs7020341 (9q33.1; P =3.04 × 10 −11 ), rs2268894 (2q24.2; P =5.89 × 10 −11 ) and rs2289881 (5q12.3; P =2.73 × 10 −8 ). We previously discovered two of the novel loci, rs7020341 and rs2268894 (ref. 24 ), but in this higher-powered analysis they now surpassed the genome-wide significance. In addition to the four novel loci, we replicated two loci associated with hippocampal volume: rs7492919 and rs17178006 (refs 23 , 24 ). Hibar et al . [22] previously reported additional support for the rs17178006 association with hippocampal volume. Each novel locus identified has unique functions and has previously been linked to diseases of the brain. Variant rs7020341 lies within an intron of the astrotactin 2 ( ASTN2 ) gene ( Fig. 2d ) which encodes for a protein involved in glial-mediated neuronal migration in the developing brain [28] . Rare deletions overlapping this locus near the 3′ end of ASTN2 have been observed in patients with autism spectrum disorder and attention-deficit/hyperactivity disorder [29] . Common variants near this site are associated with autism spectrum disorders [29] and migraine [30] . Variant rs2268894 is located in an intron of DPP4 ( Fig. 2e ) that encodes dipeptidyl peptidase IV; an enzyme regulating response to the ingestion of food [31] , and an established target of a treatment for type 2 diabetes mellitus (vildagliptin) [32] . In addition, rs2268894 is in strong LD ( r 2 =0.83) with a genome-wide significant locus associated with a decreased risk for schizophrenia (rs2909457) [33] ; however, the allele that increases risk for schizophrenia also increases hippocampal volume even though patients with schizophrenia show decreased hippocampal volume relative to controls [6] . Variant rs11979341 lies in an intergenic region ( Fig. 2c ) around 200 kb upstream of the sonic hedgehog ( SHH ) gene, crucial for neural tube formation [34] . Adult brain expression data provide some evidence that rs11979341-C increases the expression of SHH in adult human hippocampus [35] ( P =0.0089). Finally, variant rs2289881 lies within an intron of the microtubule-associated serine/threonine kinase family member 4 ( MAST4 ) gene ( Fig. 2f ). The protein product of MAST4 modulates the microtubule scaffolding; the gene has been linked to susceptibility for atherosclerosis in HIV-infected men [36] , and atypical frontotemporal dementia [37] . Effect sizes from the full sample were almost identical to those obtained from a subset meta-analysis (Pearson’s r 2 >0.99; n =22,761) that removed all patients diagnosed with a neuropsychiatric disorder. Observed effects are therefore not likely to be driven by inclusion of patients with brain disorders. All significant loci are tabulated in Table 1 . We found little evidence that these effects could be generalized to populations of African, Japanese, and Mexican-American ancestry, which could be due to the limited power from smaller non-European sample sizes available ( n =6,722; Supplementary Data 5 ). We estimated that 18.76% (s.e. 1.56%) of the variance in hippocampal volume could be explained by genotyped common genetic variation. This effect was only tested within populations of European ancestry and does not necessarily reflect the level of explained variance in other populations worldwide. This is a substantial fraction of the overall genetic component of variance determined by twin heritability studies, and the heritability of hippocampal volume is relatively high at around 70% (refs 19 , 20 , 21 ). With the same LDSCORE method, we estimated the amount of variance explained by common gene variants belonging to known functional cell categories [26] . We discovered enrichment of genomic regions conserved across mammals, which may have a strong evolutionary role in the hippocampal formation, a structure much more extensively developed in mammals than in other vertebrates [38] . Given that hippocampal atrophy is a hallmark of Alzheimer’s disease pathology [39] , we were motivated to examine common genetic overlap between hippocampal volume and Alzheimer’s disease risk. We found a significant negative relationship ( r g =−0.155 (s.e. 0.0529), P =0.0034), through which loci associated with decreased hippocampal volume also increase risk for AD. This confirms a shared etiological component between AD and hippocampal volume whereby genetic variants influencing hippocampal volume also modify the risk for developing AD. As the hippocampal formation is a complex structure comprised of diverse functional units, we sought to examine the genetic variants identified in our analysis for focal effects on hippocampal subfield volumes. When assessing 13 subfields of the hippocampus (26 total, left and right) we found that two of the top variants from our analysis (rs77956314 and rs7020341) had largely non-specific effects: most of the subfield volumes showed significant evidence of association ( Supplementary Data 8 ). The variant rs61921502 showed a lateralized effect across the body of the right hippocampal formation, which includes the DG, subiculum, CA1 and fissure. Volume losses are frequently observed across the hippocampal body in AD [40] , major depression [41] , bipolar disorder [42] and temporal lobe epilepsy [43] . Prior pathway analyses have implicated the rs61921502 with MSR3B , a gene related to oxidative stress [24] . Genetic variation at MSR3B may influence neurogenesis specifically within the dentate regions of the hippocampal body, where cell proliferation is known to continue into adulthood in healthy humans [44] . However, further functional validation is required to test this hypothesis. Finally, the variant rs2268894 was associated with volume differences in the left hippocampal tail, a subfield that has previously shown shape abnormalities [45] and volume differences [46] in schizophrenia. Here we identified four novel loci associated with hippocampal volume and examined each variant for localized effects in hippocampal subfields. When partitioning the full genome-wide association results into functionally annotated categories, we discovered that SNPs in evolutionarily conserved regions were significantly over-represented in their contribution to hippocampal volume. Further, we found significant evidence of shared genetic overlap between hippocampal volume and Alzheimer’s disease. This large international effort shows that by mapping out the genetic influences on brain structure, we may begin to derive mechanistic hypotheses for brain regions causally implicated in the risk for neuropsychiatric disorders. Subjects and sites High-resolution MRI brain scans and genome-wide genotyping data were available for 33,536 individuals from 65 sites in two large consortia: the ENIGMA Consortium and the CHARGE Consortium. Full details and demographics for each participating cohort are given in Supplementary Data 1 . All participants (or their legal representatives) provided written informed consent. The institutional review board of the University of Southern California and the local ethics board of Erasmus MC University Medical Center approved this study. Imaging analysis and quality control Hippocampal volumes were estimated using the automated and previously validated segmentation algorithms, FSL FIRST [47] from the FMRIB Software Library (FSL) and FreeSurfer [48] . Hippocampal segmentations were visually examined at each site, and poorly segmented scans were excluded. Sites also generated histogram plots to identify any volume outliers. Individuals with a volume more than three standard deviations away from the mean were visually inspected to verify proper segmentation. Statistical outliers were included in analysis if they were properly segmented; otherwise, they were removed. Average bilateral hippocampal volume was highly correlated across automated procedures used to measure it (Pearson’s r =0.74) [22] . A measure of head size—intracranial volume (ICV)—was used as a covariate in these analyses to adjust for volumetric differences due to differences in head size alone. Most sites measured ICV for each participant using the inverse of the determinant of the transformation matrix required to register the subject’s MRI scan to a common template and then multiplied by the template volume (1,948,105 mm 3 ). Full details of image acquisition and processing performed at each site are given in Supplementary Data 2 . Genetic imputation and quality control Genetic data were obtained at each site using commercially available genotyping platforms. Before imputation, genetic homogeneity was assessed in each sample using multi-dimensional scaling (MDS). Ancestry outliers were excluded by visual inspection of the first two components. The primary analysis and all data presented in this main text were derived from subjects with European ancestry. Replication attempts in subjects of additional ancestries are presented in Supplementary Data 5 . Data were further cleaned and filtered to remove single-nucleotide polymorphisms (SNPs) with low minor allele frequency (MAF<0.01), deviations from Hardy–Weinberg Equilibrium (HWE; P <1 × 10 −6 ), and poor genotyping call rate (<95%). Cleaned and filtered datasets were imputed to the 1000 Genomes Project reference panel (phase 1, version 3) using freely available and validated imputation software (MaCH/minimac, IMPUTE2, BEAGLE, GenABLE). After imputation, genetic data were further quality checked to remove poorly imputed SNPs (estimated R 2 <0.5) or low MAF (<0.5%). Details on filtering criteria, quality control, and imputation at each site may be found in Supplementary Data 3 . Genome-wide association analysis and statistical models GWAS were performed at each site, as follows. Mean bilateral hippocampal volume ((left+right)/2) was the trait of interest, and the additive dosage value of a SNP was the predictor of interest, while controlling for 4 MDS components, age, age 2 , sex, intracranial volume and diagnosis (when applicable). For studies with data collected from multiple centres or scanners, additional covariates were also included in the model to adjust for any scanning site effects. Sites with family data (NTR-Adults, BrainSCALE, QTIM, SYS, GOBS, ASPSFam, ERF, GeneSTAR, NeuroIMAGE, OATS, RSIx) used mixed-effects models to account for familial relationships, in addition to covariates stated previously. The primary analyses for this paper focused on the full set of individuals, including datasets with patients, to maximize power. We re-analysed the data excluding patients to verify that detected effects were not due to disease alone. The regression coefficients for SNPs with P <1 × 10 −5 in the model including all patients were almost perfectly correlated with the regression coefficients from the model including only healthy individuals (Pearson’s r =0.996). Full details for the software used at each site are given in Supplementary Data 3 . The GWAS of mean hippocampal volume was performed at each site, and the resulting summary statistics uploaded to a centralized site for meta-analysis. Before meta-analysis, GWAS results from each site were checked for genomic inflation and errors using Quantile–Quantile (QQ) plots ( Supplementary Figs 1 and 2 ). GWAS results from each site were combined using a fixed-effects sample size-weighted meta-analysis framework as implemented in METAL [49] . Data were meta-analysed first in the ENIGMA and CHARGE Consortia separately and then combined into a final meta-analysed result file. After the final meta-analysis, SNPs were excluded if the SNP was available for fewer than 5,000 individuals. Variance explained and genetic overlap in hippocampal volume The common genetic overlap, total variance explained by the GWAS, and the partitioned heritability analyses were estimated using LDSCORE [25] , [26] . Following from the polygenic model, an association test statistic at a given locus includes signal from all linked loci. Given a heritable polygenic trait, a SNP in high LD with, or tagging, a large number of SNPs is on average likely to show stronger association than a SNP that is not. The magnitude of information conveyed by each variant (a function of the number of SNPs tagged taking into account the strength of the tagging) is summarized as an LD score. By regressing the LD scores on the test statistics, we estimated the proportion of variance in the trait explained by the variants included in the analysis. As an extension, two LD score models for two separate traits can be used to estimate the covariance (and correlation) structure to yield an estimate of the common genetic overlap ( r g ) between any two trait pairs. Here we estimated the common genetic overlap between hippocampal volume and Alzheimer’s disease [50] . Standard errors were estimated using a block jackknife. Genomic partitioning into functional categories As well as estimating the total variance explained, the genomic heritability ( h 2 g ) can be partitioned into specific subsets of variants. The functional annotation partitioning used the pre-prepared LDSCORE and annotation (.annot) files available online (see URLs) following the method of Finucane et al . [26] . These analyses use the following 24 functional classes not specifically unique to any cell type: coding, UTR, promoter, intron, histone marks H3K4me1, H3K4me3, H3K9ac5 and two versions of H3K27ac, open chromatin DNase I hypersensitivity Site (DHS) regions, combined chromHMM/Segway predictions, regions conserved in mammals, super-enhancers and active enhancers from the FANTOM5 panel of samples (Finucane et al ., page 4) [26] . Annotated coordinates are determined by a combination of all cell types from ENCODE. As in Finucane et al . [26] , to avoid bias, we included the 500 bp windows surrounding the variants included in the functional classes. The chromosome-partitioned analyses were conducted using LDSCOREs calculated for each chromosome. Following the method of Bulik-Sullivan et al . [25] , these analyses focus on the variants within HapMap3 as these SNPs are typically well imputed across cohorts. Enrichment of a given partition is calculated as the proportion of h 2 g explained by that partition divided by the proportion of variants in the GWAS that fall into that partition. All LDSCORE analyses used non-genomic controlled meta-analyses. Gene annotation and pathway analysis Gene annotation, gene-based test statistics, and pathway analysis were performed using the KGG2.5 software package [51] ( Supplementary Data 6 and 7 ). LD was calculated based on RSID numbers using the 1000 Genomes Project European samples as a reference (see URLs). For annotation, SNPs were considered ‘within’ a gene, if they fell within 5 kb of the 3′/5′ UTR based on human genome (hg19) coordinates. Gene-based tests were performed using the GATES test [51] without weighting P values by predicted functional relevance. Pathway analysis was performed using the HYST test of association [52] . For all gene-based tests and pathway analyses, results were considered significant if they exceeded a Bonferroni correction threshold accounting for the number of pathways in the REACTOME database tested such that P thresh =0.05/(671 pathways)=7.45 × 10 −5 . Annotation of SNPs with epigenetic factors In Fig. 2 , all tracks were taken from the UCSC Genome Browser Human hg19 assembly. SNPs (top 5%) shows the top 5% associated SNPs within the locus and are coloured by their correlation to the top SNP. Genes shows the gene models from GENCODE version 19. Hippocampus gives the predicted chromatin states based on computational integration of ChIP-seq data for 18 chromatin marks in human hippocampal tissue derived from the Roadmap Epigenomics Consortium [53] . The 18 chromatin states from the hippocampus track are as follows: TssA (Active TSS), TssFlnk (Flanking Active TSS), TssFlnkU (Flanking TSS Upstream), TssFlnkD (Flanking TSS Downstream), Tx (Strong transcription), TxWk (Weak transcription), EnhG1 (Genic Enhancers 1), EnhG2 (Genic Enhancers 2), EnhA1 (Active Enhancers 1), EnhA2 (Active Enhancers 2), EnhWk (Weak Enhancers), ZNF/Rpts (ZNF genes & repeats), Het (Heterochromatin), TssBiv (Bivalent/Poised TSS), EnhBiv (Bivalent Enhancer), ReprPC (Repressed PolyComb), ReprPCWk (Weak Repressed PolyComb), Quies (Quiescent/Low). Additional information about the 18 state chromatin model is detailed elsewhere [53] . Conservation is the basewise conservation score over 100 vertebrates estimated by PhyloP from the UCSC Genome Browser Human hg19 assembly. Analysis of hippocampal subfields We segmented the hippocampal formation into 13 subfield regions: CA1, CA3, CA4, fimbria, Granule Layer+Molecular Layer+Dentate Gyrus Boundary (GC_ML_DG), hippocampal-amygdaloid transition area (HATA), hippocampal tail, hippocampal fissure, molecular layer (HP), parasubiculum, presubiculum and subiculum using a freely available, validated algorithm distributed with the FreeSurfer image analysis package [54] . We measured the hippocampal subfield volumes within the Rotterdam ( n =4,491) and HUNT ( n =877) cohorts. Volumes from the 26 subfield regions (13 in each hemisphere) were the phenotypes of interest and individually assessed for significance with the top variants from our primary analysis while correcting for the following nuisance variables: 4 MDS components, age, age 2 , sex, intracranial volume. Association statistics from each of the tests in the Rotterdam and HUNT cohorts were meta-analysed using a fixed-effects inverse variance-weighted model yielding the final results. We declare an individual test significant if the P value is less than a Bonferroni-corrected P value threshold accounting for the total number of tests: P thresh =0.05/(26 subfields × 6 SNPs)=3.21 × 10 −4 . Data availability The genome-wide summary statistics that support the findings of this study are available upon request from the corresponding authors MAI and PMT (see URLs). The data are not publicly available due to them containing information that could compromise research participant privacy/consent. URLs https://github.com/bulik/ldsc http://enigma.usc.edu/protocols/genetics-protocols/ http://gump.qimr.edu.au/general/gabrieC/LocusTrack/ http://enigma.ini.usc.edu/download-enigma-gwas-results/ http://www.internationalgenome.org/data How to cite this article: Hibar, D. P. et al . Novel genetic loci associated with hippocampal volume. Nat. Commun. 8 , 13624 doi: 10.1038/ncomms13624 (2017). Publisher’s note: Springer Nature remains neutral with regard to jurisdictional claims in published maps and institutional affiliations.